Rad54B serves as a scaffold in the DNA damage response that limits checkpoint strength The strength of the DNA damage checkpoint critically influences cell fate, yet the mechanisms behind the fine tuning of checkpoint strength during the DNA damage response (DDR) are poorly understood. Here we show that Rad54B—a SNF2 helicase-like DNA-repair protein—limits the strength of both the G1/S and G2/M checkpoints. We find that Rad54B functions as a scaffold for p53 degradation via its direct interaction with the MDM2–MDMX ubiquitin–ligase complex. During the early phases of the DDR, Rad54B is upregulated, thereby maintaining low checkpoint strength and facilitating cell cycle progression. Once the p53-mediated checkpoint is established, Rad54B is downregulated, and high checkpoint strength is maintained. Constitutive upregulation of Rad54B activity, which is frequently observed in tumours, promotes genomic instability because of checkpoint override. Thus, the scaffolding function of Rad54B dynamically regulates the maintenance of genome integrity by limiting checkpoint strength. DNA damage responses (DDRs) play critical roles in maintenance of homeostasis, as exemplified by the findings that diverse human diseases, including cancer, are caused by deficiencies in DDR components [1] . The response to DNA double-strand breaks consists of both positive and negative regulatory pathways, which transmit their signals from sensors to effectors to execute cellular responses. These pathways are composed of proteins involved in post-translational modification, such as phosphorylation and ubiquitination. Accumulating evidence suggests that scaffold-like proteins, such as those harbouring BRCT domains [2] , are involved in the signal transduction pathways of DDRs by recruiting various components and regulators. A recent study has revealed that DNA repair scaffolds directly modulate the checkpoint signalling pathway in budding yeast [3] . Therefore, the functions of scaffold-like proteins in the DDR play essential roles in the coordination of cellular responses to maintain homeostasis. Human Rad54B was initially identified as a homologue of human Rad54, a central effector of homologous recombination (HR), and mutations in its gene have been observed in primary cancers [4] . Rad54B and Rad54 belong to a subfamily of double-stranded DNA-dependent ATPases referred to as the SWI2/SNF2 family, which is characterized by conserved helicase-like sequence motifs [5] . Although previous studies suggested that Rad54B plays roles in the HR and DNA repair processes [6] , [7] , [8] , [9] , biochemical analysis has shown that Rad54B is a less active DNA-dependent ATPase than Rad54 (ref. 10 ). In addition, in contrast to Rad54, the ATPase activity of Rad54B is not enhanced by the presence of Rad51 and single-stranded DNA. These observations led us to hypothesize that Rad54B plays unknown roles aside from HR repair. During the cellular response to DNA damage, the choice between cell cycle arrest and progression is critical to the determination of the cell fate. However, despite the importance of the choice, the mechanisms by which this choice is modulated are poorly understood. Here we show that the SNF2-like domain of Rad54B serves as a scaffold for p53 degradation by facilitating MDM2–MDMX-mediated ubiquitination. Rad54B, whose levels are dynamically regulated in response to DNA damage, regulates the choice between cell cycle arrest and progression by fine-tuning the expression levels of p53. These data suggest that the scaffolding function of Rad54B plays an essential role in the coordination of cellular responses after DNA damage. Rad54B is a novel DNA damage-responsive protein First, we examined how Rad54B levels are regulated during the DDR. We found that the levels of Rad54B dynamically changed in response to the genotoxic stresses ( Fig. 1a and Supplementary Fig. 1a ). Because it appeared that the change in the levels of Rad54B negatively correlated to those of p53, we examined whether p53 is involved in the regulation of the Rad54B levels. Rad54B was transcriptionally suppressed by p53 at a late time point after DNA damage ( Fig. 1b ). In addition, the Rad54B protein and mRNA levels were suppressed by Nutlin-3-mediated p53 induction ( Fig. 1c ), suggesting that this transcriptional repression mechanism was independent of p53 modification upon DNA damage. Some p53-repressed targets are regulated by the cyclin-dependent kinase inhibitor p21 (ref. 11 ). However, the repression of Rad54B by p53 was not mediated by p21 ( Supplementary Fig. 1b ). 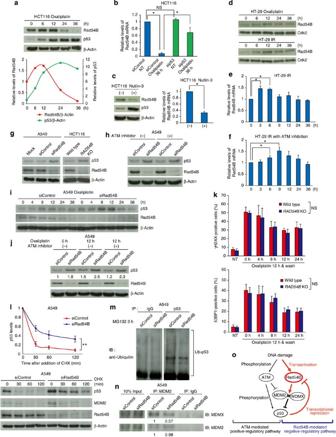Figure 1: Rad54B constitutes a novel negative-regulatory pathway for p53 independently of ATM. (a) The responses of Rad54B and p53 expression to oxaliplatin treatment in HCT116 cells harbouring wild-type p53. Quantification of each protein level is shown below. (b) The contribution of p53 to the reduction in Rad54B after DNA damage (mean±s.d.). NS, not significant; *P<0.05, two-tailedt-test,n=3. (c) The effects of DNA damage-independent p53 induction by Nutlin-3 (10 μM, 12 h) on Rad54B protein and mRNA expression (mean±s.d.). *P<0.05, two-tailedt-test,n=3. (d) Western blot for Rad54B after oxaliplatin treatment or IR of HT-29 cells harbouring mutant p53. (e,f) The Rad54B mRNA levels after IR and the effects of ATM inhibition (mean±s.d.). *P<0.05, two-tailedt-test,n=3. (g) Western blot for p53 after Rad54B inhibition. (h) The effects of ATM inhibition on Rad54B-mediated p53 inhibition. (i) Western blot for p53 after DNA damage with Rad54B inhibition. (j) The effects of ATM inhibition on Rad54B-mediated p53 inhibition during the DDR. (l) The stability of the p53 protein after cycloheximide (CHX) treatment (mean±s.e.m.;n=3). **P=0.0039, Wilcoxon matched-pairs signed-rank test. (k) The number of γH2AX and 53BP1 foci-positive cells at the indicated time points after oxaliplatin treatment and washing were counted (mean±s.d.). NS, not significant; two-tailed Welch’st-test,n=5 for each time point. (m) Western blot for ubiquitinated p53 after proteasome inhibition using MG132 (10 μM). (n) The MDM2–MDMX complex was analysed by immunoprecipitation after 6 h of proteasome inhibition using MG132 (10 μM). (o) The MDM2–MDMX-mediated ubiquitination-dependent feedback inhibitory loop between Rad54B and p53. Rad54B counteracts the canonical ATM kinase-mediated pathway during the DDR. Figure 1: Rad54B constitutes a novel negative-regulatory pathway for p53 independently of ATM. ( a ) The responses of Rad54B and p53 expression to oxaliplatin treatment in HCT116 cells harbouring wild-type p53. Quantification of each protein level is shown below. ( b ) The contribution of p53 to the reduction in Rad54B after DNA damage (mean±s.d.). NS, not significant; * P <0.05, two-tailed t- test, n =3. ( c ) The effects of DNA damage-independent p53 induction by Nutlin-3 (10 μM, 12 h) on Rad54B protein and mRNA expression (mean±s.d.). * P <0.05, two-tailed t- test, n =3. ( d ) Western blot for Rad54B after oxaliplatin treatment or IR of HT-29 cells harbouring mutant p53. ( e , f ) The Rad54B mRNA levels after IR and the effects of ATM inhibition (mean±s.d.). * P <0.05, two-tailed t- test, n =3. ( g ) Western blot for p53 after Rad54B inhibition. ( h ) The effects of ATM inhibition on Rad54B-mediated p53 inhibition. ( i ) Western blot for p53 after DNA damage with Rad54B inhibition. ( j ) The effects of ATM inhibition on Rad54B-mediated p53 inhibition during the DDR. ( l ) The stability of the p53 protein after cycloheximide (CHX) treatment (mean±s.e.m. ; n =3). ** P =0.0039, Wilcoxon matched-pairs signed-rank test. ( k ) The number of γH2AX and 53BP1 foci-positive cells at the indicated time points after oxaliplatin treatment and washing were counted (mean±s.d.). NS, not significant; two-tailed Welch’s t- test, n =5 for each time point. ( m ) Western blot for ubiquitinated p53 after proteasome inhibition using MG132 (10 μM). ( n ) The MDM2–MDMX complex was analysed by immunoprecipitation after 6 h of proteasome inhibition using MG132 (10 μM). ( o ) The MDM2–MDMX-mediated ubiquitination-dependent feedback inhibitory loop between Rad54B and p53. Rad54B counteracts the canonical ATM kinase-mediated pathway during the DDR. Full size image To investigate the mechanism underlying Rad54B induction at early time points after DNA damage, we analysed cell lines that lack functional p53 (HT-29 and H1299). Although the decreases in Rad54B expression at the late time points were not observed in these cell lines, Rad54B expression was significantly increased at the transcriptional level at the early time points ( Fig. 1d,e and Supplementary Fig. 1c–e ). We also found that this induction of Rad54B expression was independent of the activity of the ataxia-telangiectasia mutated (ATM) kinase, although the timing of this induction appeared to be delayed by ATM inhibition ( Fig. 1f and Supplementary Fig. 1f ). Thus, Rad54B is transcriptionally induced during the early phases of the DDR independently of the activity of ATM and is transcriptionally repressed as the p53 levels increase. Rad54B suppresses the p53 levels independently of ATM Although previous studies suggest that Rad54B plays roles in the HR and DNA repair processes [6] , [7] , we found a completely novel function of Rad54B; Rad54B suppressed the p53 levels and functions in the steady state independently of the activity of ATM ( Fig. 1g,h and Supplementary Fig. 1g,h ). Although MDM2 is a well-characterized negative regulator of p53, p53 upregulation was detected even though MDM2 was upregulated ( Supplementary Fig. 1g ), suggesting that MDM2 does not efficiently act as a negative regulator of p53 in the absence of Rad54B. Rad54B repressed the p53 levels and functions even after the genotoxic stresses, which was also independent of the ATM activity ( Fig. 1i,j and Supplementary Fig. 2a–c ). Interestingly, the levels of phosphorylated p53 were increased in Rad54B-knockdown cells in parallel with the p53 upregulation, whereas the upstream DDRs were not enhanced ( Supplementary Fig. 2d ). Furthermore, the amount of DNA damage during the DDR upon oxaliplatin treatment, as measured by focus formation of γH2AX or 53BP1, was not affected by Rad54B inhibition ( Fig. 1k and Supplementary Fig. 2e ). Thus, our data suggest that Rad54B inhibition upregulates the p53 levels and functions without increasing the amount of DNA damage. One previous study reported apparently contradictory results regarding the activity of p53 in Rad54/Rad54b double-knockout (KO) cells [12] . However, the findings of Mahabir et al. do not contrast with our results because of differences in the genotype of the cells used and in the experimental conditions, particularly the level of DNA damage induced. In their study, the treated cells exhibited 80% survival, whereas in our study, the treated cells exhibited 10% or less survival. The stability of the p53 protein was dramatically increased by Rad54B knockdown ( Fig. 1l and Supplementary Fig. 3a ). In addition, we detected a reduction in endogenous p53 ubiquitination in Rad54B-knockdown cells ( Fig. 1m and Supplementary Fig. 3b ). One known mechanism by which p53 is stabilized involves the alteration of the localization of the negative regulator MDM2 from the nucleus to the nucleolus [13] . We found that the MDM2 localization pattern, that is, localization predominantly in the nucleoplasm and very low expression in the nucleolus or cytoplasm, was not altered by Rad54B knockdown ( Supplementary Fig. 3c ). Another mechanism by which p53 is stabilized is the destabilization of the p53–MDM2 complex [14] . We found that the amount of MDM2 that co-immunoprecipitated with p53 was not reduced by Rad54B knockdown ( Supplementary Fig. 3d ). These data suggested that Rad54B regulates p53 via an alternative mechanism. Previous studies reported that MDMX augments the E3 ligase activity of MDM2 by forming a heterodimer with MDM2 (refs 15 , 16 ). We examined MDM2–MDMX heterodimer formation in Rad54B-knockdown cells. The amount of MDMX that bound to MDM2 was reduced by Rad54B knockdown, even after oxaliplatin treatment ( Fig. 1n and Supplementary Fig. 3e,f ), indicating that Rad54B regulates the heterodimerization between MDM2 and MDMX, thereby enhancing its ubiquitin ligase activity on p53, which we designate the Rad54B-p53 axis. Therefore, Rad54B appears to enhance the ubiquitin ligase activity of MDM2 on p53 by promoting MDM2–MDMX heterodimerization and counteracts the ATM-mediated positive regulation of p53 ( Fig. 1o ). Rad54B directly interacts with MDM2 and MDMX To clarify how Rad54B promotes MDM2–MDMX heterodimerization, we examined whether Rad54B interacts with MDM2 and MDMX. Exogenous Rad54B interacted with exogenous MDM2 and MDMX in Cos7 cells ( Fig. 2a,b ). In addition, an interaction between endogenous Rad54B and MDM2 was detected in several human cell lines, including the p53-inactive cell line HeLa ( Fig. 2c and Supplementary Fig. 4a,b ), indicating that Rad54B and MDM2 universally form a complex independent of the p53 status. We detected an interaction between endogenous Rad54B and MDMX only in the nuclear extract after proteasome inhibition, suggesting that the Rad54B–MDMX complex exists only transiently in the nucleus ( Supplementary Fig. 4c ). The findings that MDM2 knockdown does not affect the levels of Rad54B, as shown above ( Supplementary Fig. 1g ), and that Rad54B is not a substrate of proteasomal degradation ( Supplementary Fig. 4d ) indicate that the MDM2–Rad54B interaction does not reflect an enzyme–substrate interaction. 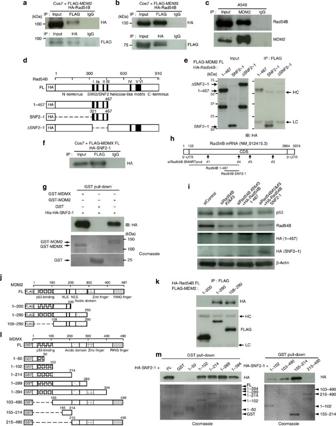Figure 2: Rad54B directly interacts with MDM2 and MDMX. (a,b) The Rad54B–MDM2 and Rad54B–MDMX interactions were detected in Cos7 cells. (c) The interaction between endogenous Rad54B and MDM2. (d) Schematic representation of Rad54B and its fragments. The seven conserved helicase-like motifs found in the SNF2 superfamily are indicated by filled boxes. (e,f) The interaction between the SNF2-1 domain and MDM2 or MDMX was confirmed by immunoprecipitation in Cos7 cells. The arrows indicate each HA-Rad54B fragment, heavy chain (HC) or light chain (LC). (g) The direct interactions were confirmed by pull-down assays. (h) Schematic representation of Rad54B mRNA and the targeting region of each siRNA. Notably, neither Rad54B 1-467 nor SNF2-1 expression was interfered using siRNA #2 or #3. (i) The effects of supplementation of the Rad54B fragments to the Rad54B-knockdown cells were analysed. (j) Schematic representation of MDM2 and its fragments. (k) The interaction between the MDM2 fragments and full-length Rad54B was analysed by immunoprecipitation in Cos7 cells. (l) Schematic representation of MDMX and its fragments. (m) The interaction between the MDMX fragment and the Rad54B SNF2-1 fragment was analysed by pull-down assays. Figure 2: Rad54B directly interacts with MDM2 and MDMX. ( a , b ) The Rad54B–MDM2 and Rad54B–MDMX interactions were detected in Cos7 cells. ( c ) The interaction between endogenous Rad54B and MDM2. ( d ) Schematic representation of Rad54B and its fragments. The seven conserved helicase-like motifs found in the SNF2 superfamily are indicated by filled boxes. ( e , f ) The interaction between the SNF2-1 domain and MDM2 or MDMX was confirmed by immunoprecipitation in Cos7 cells. The arrows indicate each HA-Rad54B fragment, heavy chain (HC) or light chain (LC). ( g ) The direct interactions were confirmed by pull-down assays. ( h ) Schematic representation of Rad54B mRNA and the targeting region of each siRNA. Notably, neither Rad54B 1-467 nor SNF2-1 expression was interfered using siRNA #2 or #3. ( i ) The effects of supplementation of the Rad54B fragments to the Rad54B-knockdown cells were analysed. ( j ) Schematic representation of MDM2 and its fragments. ( k ) The interaction between the MDM2 fragments and full-length Rad54B was analysed by immunoprecipitation in Cos7 cells. ( l ) Schematic representation of MDMX and its fragments. ( m ) The interaction between the MDMX fragment and the Rad54B SNF2-1 fragment was analysed by pull-down assays. Full size image Next, we identified the domains responsible for these interactions. Rad54B is primarily composed of three domains ( Fig. 2d ). In Cos7 cells, SNF2-1 was responsible for the interaction between Rad54B and both MDM2 and MDMX ( Fig. 2e,f ). Furthermore, the SNF2-1 protein was pulled down with the GST–MDM2 or GST–MDMX protein but not with GST alone ( Fig. 2g ), indicating that the Rad54B–MDM2 and Rad54B–MDMX interactions are direct. This domain of Rad54B is characterized by a DExH-box helicase motif and a Walker A nucleotide-binding motif [4] . Although this domain is well conserved among the members of the SWI2/SNF2 family, including Rad54, Rad54 did not interact with MDM2 ( Supplementary Fig. 4e ). Our next interest was to determine whether the ATPase activity of Rad54B plays any role in the Rad54B-p53 axis. Interestingly, the DExH-box domain of Rad54B (SNF2-1) alone was sufficient to downregulate p53 ( Fig. 2h,i ). The crystal structure studies of the SWI2/SNF2 helicase-like domains of Sulfolobus solfataricus Rad54 (SsoRad54) and zebrafish Rad54 revealed that the N-terminal half of the SWI2/SNF2 helicase-like domain (DExx-box domain) faces the C-terminal half of the SWI2/SNF2 helicase-like domain (HELICc domain) [17] , [18] . Furthermore, mutations in each domain have been shown to affect the double-stranded DNA-dependent ATPase activity of SsoRad54, indicating that both the DExx-box and HELICc domains are required for its catalytic activity [17] . Therefore, the result shown in Fig. 2i suggests that Rad54B likely regulates p53 in an ATPase activity-independent manner. Thus, the DExH-box domain of Rad54B not only contributes to the ATPase activity but also functions as an interface for protein–protein interaction. MDM2 is composed of four domains ( Fig. 2j ). With respect to the Rad54B-binding site in MDM2, deletion of the p53-binding domain, the zinc finger domain and the RING finger domain did not affect the interaction between MDM2 and Rad54B, but deletion of the acidic domain caused a loss of the interaction ( Fig. 2k ). Therefore, the acidic domain in MDM2 is responsible for its interaction with Rad54B. Some MDM2-binding partners, such as ARF and YY1, are known to bind to this domain and participate in the negative regulation of p53. However, as shown above ( Supplementary Fig. 3c,d ), the mechanism underlying the negative regulation of p53 by Rad54B is distinct from that by ARF or YY1. Because exogenous MDMX expression in cells is known to produce some artifactual results [19] , we identified the Rad54B-binding site in MDMX by pull-down assays ( Supplementary Fig. 4f ). MDMX primarily consists of four domains ( Fig. 2l ). We identified two Rad54B-binding sites located in the N-terminus of MDMX, one of which is the p53-binding domain ( Fig. 2m ). These data suggest that Rad54B can bind to MDMX independent of p53. Rad54B serves as a scaffold for MDM2–MDMX heterodimerization To determine whether the Rad54B–MDM2 and Rad54B–MDMX interactions are sufficient for the mechanism underlying the Rad54B-p53 axis, we performed an in vitro ubiquitination assay using recombinant proteins. Consistent with previous reports, MDMX enhanced the p53 polyubiquitination activity of MDM2 in vitro ( Fig. 3a , lanes 2, 4). Moreover, p53 polyubiquitination was further enhanced by adding SNF2-1 in addition to MDMX ( Fig. 3a , lanes 3–5), indicating that Rad54B plays a role in the regulation of p53 polyubiquitination by stimulating MDM2–MDMX heterodimerization and ligase activity. 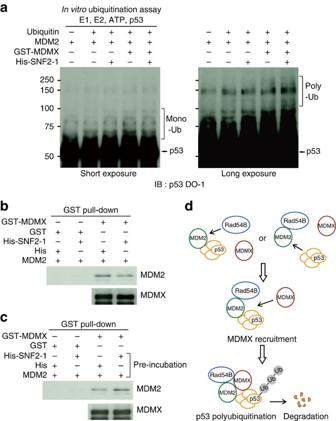Figure 3: Rad54B enhances p53 ubiquitination by recruiting MDMX to MDM2 and promoting MDM2–MDMX heterodimerization. (a)In vitroubiquitination assays for p53. (b) Pull-down assays in which all indicated proteins were included simultaneously. The western blot shown below displays the same amount of MDMX in each product. (c) Pull-down assays in which the indicated proteins were pre-incubated for 1 h. The western blot shown below displays the same amount of MDMX in each product. (d) A hypothetical model for the sequence of complex formation in the Rad54B-p53 axis. Upon p53 ubiquitination, either p53 is recruited to the Rad54B–MDM2 complex or Rad54B is recruited to the p53–MDM2 complex. After formation of the Rad54B–MDM2–p53 complex, MDMX is recruited to MDM2 by Rad54B, followed by p53 polyubiquitination and degradation. Figure 3: Rad54B enhances p53 ubiquitination by recruiting MDMX to MDM2 and promoting MDM2–MDMX heterodimerization. ( a ) In vitro ubiquitination assays for p53. ( b ) Pull-down assays in which all indicated proteins were included simultaneously. The western blot shown below displays the same amount of MDMX in each product. ( c ) Pull-down assays in which the indicated proteins were pre-incubated for 1 h. The western blot shown below displays the same amount of MDMX in each product. ( d ) A hypothetical model for the sequence of complex formation in the Rad54B-p53 axis. Upon p53 ubiquitination, either p53 is recruited to the Rad54B–MDM2 complex or Rad54B is recruited to the p53–MDM2 complex. After formation of the Rad54B–MDM2–p53 complex, MDMX is recruited to MDM2 by Rad54B, followed by p53 polyubiquitination and degradation. Full size image Next, we investigated the detailed properties of each complex by pull-down assays to further elucidate the relationship between Rad54B and the MDM2–MDMX heterodimer. As shown in Fig. 3b , when the three components GST–MDMX, MDM2 and SNF2-1 were added to the reaction simultaneously, the amount of MDM2 binding to GST–MDMX was not increased but rather was reduced, likely because SNF2-1 binds to both MDM2 and MDMX, thereby disturbing the formation of the MDM2–MDMX heterodimer. This result suggests that excess SNF2-1 disturbs MDM2–MDMX heterodimerization by preferentially forming complexes with both MDM2 and MDMX. In contrast, when MDMX was added after allowing MDM2–SNF2-1 complex formation, MDMX efficiently bound to MDM2 ( Fig. 3c ). These data suggest that Rad54B serves as a scaffold for MDM2–MDMX heterodimerization by recruiting MDMX to MDM2 and facilitates efficient p53 degradation ( Fig. 3d ). Rad54B promotes mutagenic adaptation to the G2/M checkpoint To determine the relevance of Rad54B-mediated p53 regulation in cell fate determination after DNA damage, we investigated the cell cycle distribution after induction of DNA damage. We found that the number of cells in the G2/M phase was increased in RAD54B KO HCT116 cells after oxaliplatin treatment ( Fig. 4a ) and in RAD54B KO HCT116 and Rad54B-knockdown A549 cells after ionizing radiation (IR; Supplementary Fig. 5a,b ). In addition, we confirmed that the phenotype of increased G2/M arrest in RAD54B KO cells was rescued by introducing green fluorescent protein (GFP)-conjugated Rad54B ( Fig. 4b and Supplementary Fig. 5c ). Interestingly, the increase in G2/M-arrested RAD54B KO cells after oxaliplatin treatment was dependent on the p53 levels ( Fig. 4c ). These findings indicated that the G2/M checkpoint strength is reduced by the Rad54B-p53 axis. Notably, aneuploidy was increased by oxaliplatin treatment in wild-type HCT116 cells ( Fig. 4a ). In addition, the number of RAD54B KO cells in sub-G1 was decreased after oxaliplatin treatment ( Fig. 4a ). We confirmed that this result was due to a reduction in apoptotic cells ( Supplementary Fig. 5d ). Therefore, because most RAD54B KO cells are strongly arrested at the G2 phase, aneuploidy or apoptosis arising after release from this arrest appears to be decreased. 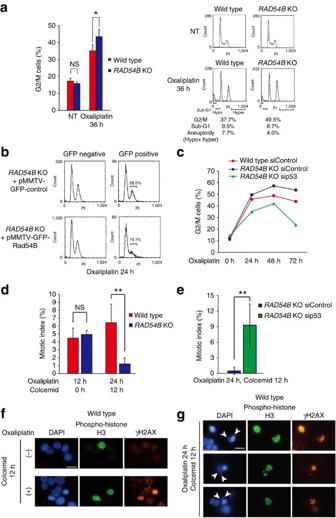Figure 4: Rad54B promotes mutagenic adaptation by dampening p53-dependent G2/M checkpoint maintenance. (a) The number of the cells in the G2/M phase after oxaliplatin treatment (mean±s.e.m.;n=3). Representative diagrams are shown in the right panel. NS, not significant; *P=0.019, two-tailed pairedt-test. (b) The cell cycle distributions of the cells transfected with the indicated constructs were analysed by flow cytometry. The diagrams shown are representative of three independent experiments. (c) The number of G2/M-phase p53-knockdownRAD54BKO cells after oxaliplatin treatment was measured at the indicated time points. The graph shown is representative of four independent experiments. (d) The oxaliplatin-treated cells were supplemented with colcemid (0.1 μg ml−1) 12 h before measurement of the mitotic index (mean±s.d.). NS, not significant; **P<0.001, two-tailed Welch’st-test,n=5. (e) p53-knockdownRAD54BKO cells were analysed as ind(mean±s.d.). **P<0.001, two-tailed Welch’st-test,n=10. (f,g) The oxaliplatin-treated wild-type cells were supplemented with colcemid 12 h before fixation and stained with phospho-histone H3 (a mitosis marker) and γH2AX (a DNA damage marker). A representative field is shown. Scale bar, 10 μm. The arrows indicate the fragmentation of chromosomes. Figure 4: Rad54B promotes mutagenic adaptation by dampening p53-dependent G2/M checkpoint maintenance. ( a ) The number of the cells in the G2/M phase after oxaliplatin treatment (mean±s.e.m. ; n =3). Representative diagrams are shown in the right panel. NS, not significant; * P =0.019, two-tailed paired t- test. ( b ) The cell cycle distributions of the cells transfected with the indicated constructs were analysed by flow cytometry. The diagrams shown are representative of three independent experiments. ( c ) The number of G2/M-phase p53-knockdown RAD54B KO cells after oxaliplatin treatment was measured at the indicated time points. The graph shown is representative of four independent experiments. ( d ) The oxaliplatin-treated cells were supplemented with colcemid (0.1 μg ml −1 ) 12 h before measurement of the mitotic index (mean±s.d.). NS, not significant; ** P <0.001, two-tailed Welch’s t- test, n =5. ( e ) p53-knockdown RAD54B KO cells were analysed as in d (mean±s.d.). ** P <0.001, two-tailed Welch’s t- test, n =10. ( f , g ) The oxaliplatin-treated wild-type cells were supplemented with colcemid 12 h before fixation and stained with phospho-histone H3 (a mitosis marker) and γH2AX (a DNA damage marker). A representative field is shown. Scale bar, 10 μm. The arrows indicate the fragmentation of chromosomes. Full size image As for inactivation of the G2/M checkpoint, previous studies showed that some cells with unrepaired DNA damage escape from the G2/M checkpoint and enter the next cell cycle phase. This process of overriding the G2/M checkpoint, referred to as adaptation, was first described in Saccharomyces cerevisiae [20] and was recently observed in higher eukaryotes, including Xenopus cells [21] and even human cancer cells [22] . Thus, we examined whether the Rad54B-dependent abrogation of the G2/M checkpoint observed in wild-type HCT116 cells was accompanied with the cells which undergo adaptation. First, as shown in Fig. 4d , the number of RAD54B KO cells that underwent G2/M transition from 12 to 24 h after oxaliplatin addition was significantly reduced, consistent with the results in Fig. 4a , and this phenotype was rescued by p53 knockdown ( Fig. 4e ). Next, we examined whether the G2/M transition observed in wild-type cells was accompanied with DNA damage. Surprisingly, approximately 30 to 40% of the wild-type cells in mitosis displayed rigid γH2AX foci when treated with oxaliplatin ( Fig. 4f ). Furthermore, we found that adaptation was frequently accompanied by chromosomal fragmentation ( Fig. 4g ). Such fragmentation is highly mutagenic because it can lead to micronucleus formation and loss or translocation of chromosomes. These data suggest that the absolute number of cells which undergo adaptation is increased by Rad54B-mediated inactivation of the G2/M checkpoint. Overall, our data suggest that Rad54B induces highly mutagenic chromosome instability by promoting adaptation. Rad54B limits the strength of the G1/S checkpoint Next, we assessed cell morphology after treatment with genotoxic drugs for approximately 1 week ( Fig. 5a ). After oxaliplatin treatment, the RAD54B KO cells were more likely to remain attached to the dish without any appearance of cell division. 5-fluorouracil (5-FU) treatment produced similar results, except that evident and countable colonies were not formed after 5-FU treatment. Based on this finding, we hypothesized that Rad54B regulates the strength of the G1/S checkpoint as well as that of the G2/M checkpoint. Indeed, the strength of the G1/S checkpoint after 5-FU or oxaliplatin treatment was increased by RAD54B KO in HCT116 cells ( Fig. 5b and Supplementary Fig. 6a ) and by Rad54B knockdown in LoVo cells ( Supplementary Fig. 6b ), which appeared to be partially attributed to the upregulation of the cyclin-dependent kinase inhibitor p21 ( Supplementary Fig. 6c ). Notably, aneuploidy was increased by 5-FU treatment in wild-type HCT116 cells ( Fig. 5b ). Furthermore, we detected a decrease in the intake of nucleotides in RAD54B KO cells approximately 48 h after the initiation of 5-FU treatment ( Supplementary Fig. 6d ). Importantly, the phenotype of the decrease in the number of S-phase cells was rescued by p53 knockdown in RAD54B KO cells ( Fig. 5c ), suggesting that the Rad54B-p53 axis plays critical roles in the regulatory mechanism responsible for inactivation of the G1/S checkpoint. 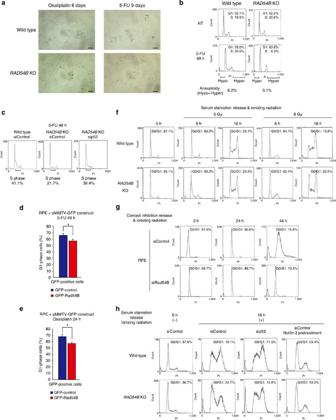Figure 5: Rad54B loosens the DNA damage-induced G1/S checkpoint. (a) Cell morphology on the indicated day after oxaliplatin or 5-FU treatment. A representative field is shown. Scale bar, 150 μm. (b) The cell cycle distributions after 5-FU treatment. The ranges of aneuploid cells are shown below the diagrams. The results are representative of three independent experiments. (c) The number of S phase p53-knockdown cells after 5-FU treatment was measured. The results are representative of three independent experiments. (d,e) The number of G1-arrested cells after DNA damage in Rad54B-overexpressing RPE cells was measured (mean±s.e.m.;n=3). *P<0.05, two-tailedt-test. (f) Serum-starvedRAD54BKO cells were released from cell cycle arrest by serum addition immediately after IR. The cell cycle distributions were analysed at the indicated time points. The results are representative of four independent experiments. (g) Fully confluent Rad54B-knockdown RPE cells were reseeded at low density immediately after IR. The cell cycle distributions were analysed at the indicated time points. The results are representative of three independent experiments. (h) Nutlin-3 was added 8 h before IR and serum addition. The cell cycle distributions were analysed at the indicated time points. The results are representative of three independent experiments. Figure 5: Rad54B loosens the DNA damage-induced G1/S checkpoint. ( a ) Cell morphology on the indicated day after oxaliplatin or 5-FU treatment. A representative field is shown. Scale bar, 150 μm. ( b ) The cell cycle distributions after 5-FU treatment. The ranges of aneuploid cells are shown below the diagrams. The results are representative of three independent experiments. ( c ) The number of S phase p53-knockdown cells after 5-FU treatment was measured. The results are representative of three independent experiments. ( d , e ) The number of G1-arrested cells after DNA damage in Rad54B-overexpressing RPE cells was measured (mean±s.e.m. ; n =3). * P <0.05, two-tailed t- test. ( f ) Serum-starved RAD54B KO cells were released from cell cycle arrest by serum addition immediately after IR. The cell cycle distributions were analysed at the indicated time points. The results are representative of four independent experiments. ( g ) Fully confluent Rad54B-knockdown RPE cells were reseeded at low density immediately after IR. The cell cycle distributions were analysed at the indicated time points. The results are representative of three independent experiments. ( h ) Nutlin-3 was added 8 h before IR and serum addition. The cell cycle distributions were analysed at the indicated time points. The results are representative of three independent experiments. Full size image Proliferation under DNA-damaged conditions increases the probability of genomic instability and mutagenesis. Thus, we examined the impact of Rad54B overexpression on the normal cell line RPE and found that Rad54B overexpression reduced the p53 levels after 5-FU or oxaliplatin treatment ( Supplementary Fig. 6e,f ). Furthermore, the number of G1-arrested RPE cells after either 5-FU or oxaliplatin treatment was reduced by introduction of the GFP–Rad54B protein ( Fig. 5d,e ). These data suggest that Rad54B overexpression in normal cells limits the G1/S checkpoint strength, thereby promoting cell cycle progression under DNA-damaged conditions. To further investigate the roles of Rad54B in the G1/S transition, we examined cells synchronized in the G0/G1 phase by serum starvation or contact inhibition. As expected, cell cycle progression after IR was delayed in G0/G1 phase-synchronized RAD54B KO HCT116 and Rad54B-knockdown RPE cells ( Fig. 5f,g and Supplementary Fig. 6g ). Furthermore, the G1/S checkpoint strength after IR was dependent on the p53 levels ( Fig. 5h ), supporting our hypothesis that the Rad54B-p53 axis regulates the G1/S checkpoint strength. Rad54B is a possible therapeutic target for cancer Based on in vitro colony formation assays, we found that the wild-type cells formed more colonies than the RAD54B KO cells ( Fig. 6a ). These data suggest that the reduction of the checkpoint strength by Rad54B confers a chance of long-term cell survival. To investigate this effect in vivo , we employed a xenograft model using nude mice. The RAD54B KO cell-derived xenografts grew more slowly than the wild-type cell-derived xenografts after either oxaliplatin or 5-FU treatment ( Fig. 6b ). Furthermore, the number of S-phase cells was reduced in RAD54B KO cell-derived xenografts compared with the wild-type cell-derived xenografts ( Fig. 6c ), suggesting that G1/S checkpoint regulation affects xenograft growth. Therefore, Rad54B inhibition enhances the sensitivity of tumour to genotoxic drugs. 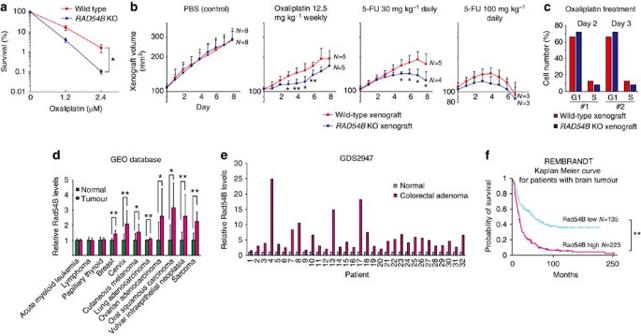Figure 6: Inhibition of Rad54B expression is a feasible strategy for cancer therapy. (a) Colony formation assays after oxaliplatin treatment (mean±s.e.m.;n=4). *P=0.0117, two-way analysis of variance with repeated measures on the log-transformed cell count,F1,3=30.4. (b) The xenograft volume after drug injection was analysed (mean±s.d., a semi-log scale). The number of mice observed is shown at the right of each line. *P<0.05, **P<0.01, two-tailed Welch’st-test on the log-transformed rate of xenograft volume growth. (c) The cell cycle distributions of the representative xenografts at the indicated time points were analysed. (d) The Rad54B levels in the neoplastic samples (means±s.d.). The number of samples analysed is shown inSupplementary Table 1. The average Rad54B levels in tumour samples were normalized to those in normal samples. *P<0.05, **P<0.01, Mann–WhitneyU-test. (e) The paired Rad54B expression data between normal and colorectal adenoma samples from the same patient. See alsoSupplementary Table 1. (f) The survival data sets from REMBRANDT. Elevated expression was defined as a twofold or greater increase in Rad54B expression. The points in the graph correspond to the censored cases. For a detailed description, see the REMBRANDT website. **P<0.001, log-rank test. Figure 6: Inhibition of Rad54B expression is a feasible strategy for cancer therapy. ( a ) Colony formation assays after oxaliplatin treatment (mean±s.e.m. ; n =4). * P =0.0117, two-way analysis of variance with repeated measures on the log-transformed cell count, F 1,3 =30.4. ( b ) The xenograft volume after drug injection was analysed (mean±s.d., a semi-log scale). The number of mice observed is shown at the right of each line. * P <0.05, ** P <0.01, two-tailed Welch’s t- test on the log-transformed rate of xenograft volume growth. ( c ) The cell cycle distributions of the representative xenografts at the indicated time points were analysed. ( d ) The Rad54B levels in the neoplastic samples (means±s.d.). The number of samples analysed is shown in Supplementary Table 1 . The average Rad54B levels in tumour samples were normalized to those in normal samples. * P <0.05, ** P <0.01, Mann–Whitney U -test. ( e ) The paired Rad54B expression data between normal and colorectal adenoma samples from the same patient. See also Supplementary Table 1 . ( f ) The survival data sets from REMBRANDT. Elevated expression was defined as a twofold or greater increase in Rad54B expression. The points in the graph correspond to the censored cases. For a detailed description, see the REMBRANDT website. ** P <0.001, log-rank test. Full size image Finally, we investigated the contribution of Rad54B to the neoplastic process. We selected data sets from the Gene Expression Omnibus database provided by NCBI ( http://www.ncbi.nlm.nih.gov/geo/ ) and used these data to compare the expression levels of Rad54B between normal and tumour samples. As shown in Fig. 6d , Rad54B expression was elevated in many different types of solid tumours. In addition, the two data sets that provided paired expression data between normal and neoplastic samples from the same patient revealed that all of the samples from colorectal adenoma and 80% of the samples from lung squamous carcinoma displayed elevated Rad54B expression ( Fig. 6e and Supplementary Table 1 ). Notably, enhanced Rad54B expression was observed even in the early stage of the neoplastic process. Furthermore, brain tumour patients displaying elevated Rad54B expression exhibited extremely poor prognosis according to the Kaplan–Meier curve analysis using the REpository for Molecular BRAin Neoplasia DaTa (REMBRANDT; Fig. 6f ; http://caintegrator.nci.nih.gov/rembrandt/ ). Therefore, these results suggested that elevated Rad54B expression exacerbates clinical outcomes. Our model shown above suggests that the association between elevated Rad54B expression and the neoplastic process may be dependent on p53 protein function. However, unfortunately, none of the above databases includes any information regarding the mutation status. Therefore, according to a previous study [23] , we predicted the mutation status of the samples based on their gene expression patterns, as described in detail in the Methods section. We examined breast cancer (GDS2250), colon adenoma (GDS2947) and glioblastoma (REMBRANDT) samples and found no significant association between the predicted p53 status and the Rad54B expression pattern ( Supplementary Figs 7–9 , Supplementary Tables 2–4 ). Overall, these database analyses indicate that the Rad54B-p53 axis plays critical roles in the neoplastic process. Upon DNA damage, the sequential recruitment and activation of the DDR proteins ensure the proper choice of cell fate [1] . The timing of activation of each DDR protein varies from a few minutes to a few days after DNA damage. For example, the recruitment of the DNA-damage marker γH2AX peaks within a few hours after DNA damage, whereas the accumulation of p53 peaks at later time points. Therefore, it has been assumed that negative-regulatory mechanisms for the DDR during its early phases play a role in the coordination of cellular responses [24] . In this study, we demonstrated that the DNA damage-responsive scaffold protein Rad54B constitutes the ATM-independent negative-regulatory DDR pathway; Rad54B is upregulated during the early phases of the DDR to limit p53 activation and is downregulated during the late phases of the DDR to stably induce p53-mediated responses ( Fig. 1o ). This transcription- and ubiquitination-dependent signalling, in parallel with the phosphorylation-mediated signalling regulated by ATM, causes the latency of p53-mediated checkpoint activation ( Fig. 7a ). Imbalanced upregulation of Rad54B function promotes genomic instability via G1/S checkpoint override and adaptation to the G2/M checkpoint ( Fig. 7b ). Our discovery of this exquisite mechanism of p53 regulation via the scaffolding function of Rad54B provides the potential for a novel cancer therapy. Inhibition of Rad54B upregulates the p53 levels without increasing apoptosis even after treatment with genotoxic drugs ( Supplementary Fig. 10 ). In addition, we emphasized the potential advantages of Rad54B inhibition-mediated therapy for targeting tumours at the earlier stages of the neoplastic process ( Figs 5d,e and 6e ). Thus, Rad54B inhibition, in combination with administration of DNA-damaging agents, may represent a feasible intervention for p53-reactivating cancer therapy. 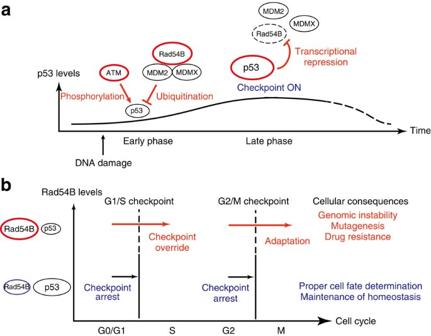Figure 7: Schematic summary of this study in terms of the time course and cell cycle. (a) The scaffold protein Rad54B causes the latency of p53-mediated checkpoint activation. During the early phases of the DDR, Rad54B constitutes the ATM-independent negative-regulatory DDR pathway. (b) The Rad54B-p53 axis regulates the checkpoint strength. Elevated expression of Rad54B induces checkpoint override, thereby enhancing genomic instability, mutagenesis and drug resistance. Figure 7: Schematic summary of this study in terms of the time course and cell cycle. ( a ) The scaffold protein Rad54B causes the latency of p53-mediated checkpoint activation. During the early phases of the DDR, Rad54B constitutes the ATM-independent negative-regulatory DDR pathway. ( b ) The Rad54B-p53 axis regulates the checkpoint strength. Elevated expression of Rad54B induces checkpoint override, thereby enhancing genomic instability, mutagenesis and drug resistance. Full size image Although the association between the checkpoint strength and cellular consequences is complex, we assumed that it primarily depends on the type of DNA damage. As shown in this study, Rad54B broadly limits the checkpoint strength regardless of the cell type and the type of DNA damage ( Figs 4a and 5b,d–g , Supplementary Fig. 5a,b and 6b ). On the other hand, the long-term cell survival rate varies depending on the type of DNA damage; RAD54B KO cells are slightly resistant to IR [6] , but they are sensitive to oxaliplatin or 5-FU treatment ( Fig. 6a–c ). Cell cycle progression under DNA-damaged conditions results in cell death in most cases, but in some cases, it confers a chance of cell survival. These contradicting aspects of cell cycle progression after DNA damage appear to explain these apparently contradicting results. As for the biological significance of limiting the checkpoint strength, we speculated that some types of DNA damage, such as that caused by an imbalance of the nucleotide pool or DNA cross-linking, might not be repaired during checkpoint arrest because such ‘potential’ DNA damage does not manifest until the cell cycle progresses to proliferative phases. Therefore, the repair protein Rad54B likely contributes to the mechanism for cell cycle progression to enable this dormant damage to manifest and to be repaired. Overall, the scaffolding function of Rad54B, by limiting the checkpoint strength, coordinates cell fate determination during the DDR. Cell culture and antibodies All cell lines were cultured in a 37 °C incubator at 5% CO 2 . The A549 and RPE cells were obtained from RIKEN Cell Bank and Clontech, respectively. The U2OS, HCT116 and H1299 cells were obtained from American Type Culture Collection. The HT-29, HCT116 cells, and their derivatives were cultured in McCoy’s 5A medium. The RPE cells were cultured in DMEM/F-12 medium. The H1299 cells were cultured in RPMI-1640 medium. All other cell lines were cultured in DMEM medium. All media were supplemented with 10% fetal bovine serum. The RAD54B KO HCT116 cells were previously described [6] . MG132 (C2211) and cycloheximide (C4859) were obtained from Sigma-Aldrich. Oxaliplatin and 5-FU were obtained from Wako. Nutlin-3 and the ATM inhibitor were obtained from Millipore. For irradiation, an X-ray generator (Pantak HF 350: Shimadzu) was used. For synchronization in the G0/G1 phase, the cells were cultured in serum-free medium for 2 days. The antibodies used in this study are shown in Supplementary Table 5 . Plasmids The plasmids for FLAG-tag or HA-tag fusion were generated by annealing oligonucleotides and ligating these regions to pcDNA3.1/Zeo or pEF4/His (Invitrogen), respectively. The plasmid for GFP fusion was generated by PCR amplification followed by cloning into the MMTV promoter-based plasmid. The plasmids for full-length human Rad54B and Rad54 were previously described [25] . The plasmid for flow cytometric analyses was generated by inserting the Rad54B-coding region into the pIRES2-EGFP vector (Clontech). The plasmids encoding full-length human MDM2, MDMX or p53 were cloned by PCR from HEK293 or RPE cell cDNA. The Rad54B, MDM2 or MDMX fragment expression plasmids were generated by PCR. The sequences of all PCR products were confirmed. For GST-tagged or 6 × His-tagged proteins, the coding sequence of each protein was ligated to pGEX-5X (GE Healthcare) or pET32a (Novagen), respectively. Plasmid transfection, immunoprecipitation and western blot The cells were transfected with the indicated plasmids using Lipofectamine 2000 reagent (Invitrogen) according to the manufacturer’s instructions. For western blot, the cells were harvested in lysis buffer (0.5% NP-40, 50 mM Tris–HCl (pH 7.4), 150 mM NaCl, 0.5 mM EDTA, 1 mM dithiothreitol, 1 mM phenylmethylsulphonyl fluoride, 10 μg ml −1 aprotinin, 50 nM cantharidin and 5 nM Microcystin-LR). For immunoprecipitation, the indicated antibody was added to the lysate, and the solution was continuously rotated at 4 °C. After 2 h, the solution was supplemented with Protein G agarose (Invitrogen) and rotated for another 1 h. The beads were washed three times with lysis buffer and denatured by boiling in SDS sample buffer. The denatured proteins were resolved by SDS–polyacrylamide gel electrophoresis and transferred to polyvinylidene difluoride membrane (Millipore). Immunoblots were detected using ECL (GE Healthcare), and the band intensity on the film was quantified using Image J software. Full scans of the blots are shown in Supplementary Figs 11 and 12 . mRNA extraction and quantitative reverse transcription–PCR Total RNA was extracted using RNAiso Plus (Takara) according to the manufacturer’s instructions. Extracted RNA was reverse-transcribed using Moloney murine leukemia virus reverse-transcriptase, ribonuclease inhibitor and random hexamers (Takara). The synthesized cDNAs were analysed for each gene expression level by real-time PCR using a Smart Cycler PCR system and SYBR Premix Ex Taq (Takara) according to the manufacturer’s instructions. The results were quantified relative to a calibration curve for each primer set and were normalized to the glyceraldehyde 3-phosphate dehydrogenase levels. All measurements were performed in triplicate. The following primers were used in this study: glyceraldehyde 3-phosphate dehydrogenase, 5′-GCACCGTCAAGGCTGAGAAC-3′ (forward) and 5′-ATGGTGGTGAAGACGCCAGT-3′ (reverse); Rad54B, 5′-TCCAGGTCTGAATGAAGAGATTAC-3′ (forward) and 5′-TCTAGTACTTTCTTCACTAGGCAG-3′ (reverse); p53, 5′-AGATGTTCCGAGAGCTGAATGAG-3′ (forward) and 5′-GAGAATGTCAGTCTGAGTCAGGC-3′ (reverse); MDM2, 5′-CCTTAGCTGACTATTGGAAATGC-3′ (forward) and 5′-ACATCAAAGCCCTCTTCAGCTTG-3′ (reverse); p21, 5′-GACTCTCAGGGTCGAAAACGG-3′ (forward) and 5′-GCGGATTAGGGCTTCCTCTTG-3′ (reverse) and Bax, 5′-ACTCCCCCCGAGAGGTCTT-3′ (forward) and 5′-GCAAAGTAGAAAAGGGCGACAA-3′ (reverse). Short interfering RNA (siRNA) All siRNAs were purchased from Dharmacon. Each siRNA (final concentration of 50–75 nM) was transfected into cells using DharmaFECT4 transfection reagent (Dharmacon). For co-transfection of siRNAs and plasmid, siRad54B #2&#3 (final concentration of 40 nM each) and pEF-HA-Rad54B 1-467 or SNF2-1 plasmid were transfected using DharmaFECT Duo transfection reagent (Dharmacon) according to the manufacturer’s instructions. Production of recombinant proteins The GST fusion proteins were expressed in E. coli BL21 cells (GE Healthcare, New England BioLabs) and were purified on an Immobilized Glutathione Column (Thermo Scientific) or Glutathione Sepharose 4B (GE Healthcare) according to the manufacturer’s instructions. The 6 × His fusion proteins were expressed in BL21(DE3) cells (Invitrogen) and were purified on a TALON resin and a TALON Disposable Gravity Column (Clontech). All proteins were dissolved in binding buffer (20 mM Tris–HCl (pH 7.4), 10 mM NaCl and 1 mM MgCl 2 ) using Amicon Ultra-0.5 10 K (Millipore). If required, the GST tag was removed using Factor Xa (New England BioLabs). GST pull-down assay For the GST pull-down assays, the indicated proteins were mixed and incubated at room temperature. After 1–2 h, the GST-tagged proteins were pulled down using Glutathione Sepharose 4B (GE Healthcare) and were eluted in elution buffer (50 mM Tris–HCl (pH 8.0) and 10 mM glutathione). The products were resolved by SDS–polyacrylamide gel electrophoresis and immunoblotted using the indicated antibody. In vitro ubiquitination assay In vitro ubiquitination assays were conducted in reaction buffer (50 mM Tris–HCl (pH 7.4), 5 mM MgCl 2 , 2 mM ATP and 2 mM dithiothreitol) supplemented with human UBE1 (6 nM), human UbcH5b (100 nM; Boston Biochem), in vitro translated p53 (0.3 μl; Promega) and MDM2 (100 ng), in the absence or presence of ubiquitin (25 μM; Boston Biochem), GST-MDMX (200 ng) and His-SNF2-1 (200 ng) at 37 °C for 2 h. The reaction was halted by adding SDS sample buffer, and the products were analysed by western blot. Cell cycle analysis Cells detached using Trypsin-EDTA were fixed if indicated and were stained using a CycleTEST PLUS DNA Reagent Kit (Becton Dickinson) according to the manufacturer’s instructions. Cell cycle analysis was performed using an EPICS XL flow cytometer (Beckman Coulter). For the 5-ethynyl-2′-deoxyuridine (EdU) assay, EdU (Invitrogen; 10 μM) was added to the medium at the indicated time before harvesting. The harvested cells were fixed in 4% paraformaldehyde for 10 min and were permeabilized using 0.5% Triton-X for 5 min at room temperature. After several washes, the incorporated EdU was labelled for 30 min by a click chemistry reaction in buffer containing 100 mM Tris–HCl (pH 8.0), 1 mM CuSO 4 and 10 μM Alexa 488 azide (Invitrogen) supplemented with 100 mM ascorbic acid. The labelled cells were stained with propidium iodide (PI) and were analysed as described above. Immunofluorescence The cells cultured on coverslips or detached using Trypsin-EDTA were fixed in 4% paraformaldehyde for 10 min at room temperature. The cells were permeabilized using 0.5% Triton-X and 0.1% SDS for 5 min, followed by blocking with 10% horse serum for 30 min. Then, the cells were incubated in primary antibodies and, subsequently, in secondary antibodies at 37 °C for 30 min. For the cells on coverslips, the cells were counterstained with 4',6-diamidino-2-phenylindole (DAPI) and mounted. Representative images were captured using an Olympus BX51 fluorescence microscope and an Olympus DP 70 digital camera equipped with an Olympus DP controller and DP manager software (Olympus). For the detached cells, the cells were analysed using a FACSAria II cell sorter (Becton Dickinson). Colony formation assay The wild-type or RAD54B KO HCT116 cells were seeded at a density of 6.0 × 10 3 cells per 60 mm dish and were treated with oxaliplatin at the indicated dose. After 7–10 days, the cells were fixed and stained to count the colonies. All measurements were performed in triplicate. Xenograft model All animal experiments were approved by the Institutional Animal Experiment Committee of the University of Tokyo. Male BALB/c SIc-nu/nu mice (4 weeks of age) were purchased from Nihon SLC (Shizuoka). Then, 2.5 × 10 6 wild-type HCT116 cells or their derivatives were injected subcutaneously. When the tumours reached approximately 100 mm 3 (Day 0), the mice were intraperitoneally injected with oxaliplatin weekly or 5-FU daily at the indicated dose. Tumour growth was measured every day after initiation of treatment, and the tumour volume was calculated as 0.5 × length × width 2 . For cell cycle analysis, the oxaliplatin-treated mice were euthanized on day 2 or 3, and the tumours were homogenized for PI staining, which was performed as described above. Analysis of the databases Using the raw expression data provided by the GEO database, the average and standard deviation of the Rad54B expression levels in normal and tumour samples were calculated and were compared using the Mann–Whitney U -test. The average Rad54B expression levels in tumour samples were normalized to those in normal samples. The gene data sets for p53 mutation status prediction were identified according to the procedure described in a previous study [23] with some modifications. Briefly, using the gene expression data provided by TCGA, the differentially expressed genes between the samples harbouring wild-type and mutant p53 were identified by excluding those genes displaying a P -value on Welch’s t -test >0.001 and by ranking the included genes in decreasing order of the log ratio. For hierarchical cluster analyses, the gene expression values were mean-centred, and the genes and the samples were clustered by Pearson correlation and average linkage (Cluster 3.0 software) to confirm the efficiency of the prediction. The clustering results were visualized using Java TreeView software. The samples from GEO or REMBRANDT were assigned to the appropriate cluster using the nearest neighbour algorithm according to the Pearson correlation-based similarity. How to cite this article: Yasuhara, T. et al. Rad54B serves as a scaffold in the DNA damage response that limits checkpoint strength. Nat. Commun. 5:5426 doi: 10.1038/ncomms6426 (2014).